Tip-enhanced nano-Raman analytical imaging of locally induced strain distribution in carbon nanotubes Tip-enhanced Raman scattering microscopy is a powerful technique for analysing nanomaterials at high spatial resolution far beyond the diffraction limit of light. However, imaging of intrinsic properties of materials such as individual molecules or local structures has not yet been achieved even with a tip-enhanced Raman scattering microscope. Here we demonstrate colour-coded tip-enhanced Raman scattering imaging of strain distribution along the length of a carbon nanotube. The strain is induced by dragging the nanotube with an atomic force microscope tip. A silver-coated nanotip is employed to enhance and detect Raman scattering from specific locations of the nanotube directly under the tip apex, representing deformation of its molecular alignment because of the existence of local strain. Our technique remarkably provides an insight into localized variations of structural properties in nanomaterials, which could prove useful for a variety of applications of carbon nanotubes and other nanomaterials as functional devices and materials. Plasmonics has recently been a rapidly growing research field in nanophotonics. It covers a wide range of applications including nanoscale circuits [1] , [2] , [3] , cancer therapy [4] , holography [5] , efficient solar cells [6] , metamaterial devices [7] , [8] , [9] , single-molecule detection [10] , [11] , biosensing [12] and nanoresolution imaging [13] . Some of the functions of surface plasmon polaritons utilized in plasmonic techniques are field enhancement, photon nanoconfinement and spectral tunability. As an application of plasmonics in nanoimaging, metallic probes have been utilized to localize photons [14] , which, when combined with Raman scattering [15] , [16] , fluorescence [17] and infrared absorption [18] spectroscopies, can provide images of the distribution of molecules at a spatial resolution typically of the order of 10~20 nm. Recently, reproducibility in imaging has been greatly improved by optimizing the fabrication methods of probe tips [19] , [20] . The oxidization of silicon, which is the base material for silver-coated cantilevers, increases the Raman scattering enhancement [19] , and template stripping of gold pyramids makes mass production of probes possible [20] . Plasmonic probes can be used for imaging the distribution of multiple components or molecular distributions within nanomaterials through fluorescence or Raman scattering spectroscopy. Images of DNA molecules [21] , carbon nanotubes (CNTs) [22] , [23] , silicon devices [24] , [25] and dye molecules [26] have been observed with tip-enhanced Raman scattering (TERS) microscopy. Recently, a single-porphyrin molecule was imaged with TERS under ultrahigh vacuum and low temperature [27] . In particular, the imaging of CNTs with variations in the number of walls, diameter, chirality, local defects and local strain is of great interest for nanomaterial scientists and nanodevice researchers. CNTs have proven their supremacy in various high-end fundamental research and practical applications, and have attracted a variety of investigations in nanoscience [28] , [29] , [30] , [31] , [32] . Many of these applications, such as electronic and optical devices, require specific positioning of the nanotubes, for example, between two electrodes. Some researchers have used atomic force microscopy (AFM) to physically manipulate CNTs with nanoscale precision [33] , [34] , [35] , [36] . This process often develops local strain in the nanotubes. Although AFM-induced strains have been observed via confocal Raman spectroscopy with diffraction-limited spatial resolution [37] , [38] , [39] , [40] , it has not been easy to investigate the localized nature of such strains that can be confined within nanoscale region, which can significantly affect the device performance. In this study, we develop localized strain in a very controlled manner in an isolated CNT and then study its distribution along the length of the nanotube, as well as its localization, by means of plasmonic nanoimaging. We employ a silver-coated nanotip to enhance and detect Raman scattering directly from a specific location of the CNT right under the apex of the tip. By scanning the tip, we are then able to construct images based on the measured local spectral shifts. The strain within a CNT, resting horizontally on a substrate, is induced by dragging the nanotube locally with a horizontal push through the apex of an AFM tip. By locally dragging a straight nanotube in a controlled manner, we are able to manipulate it into any desired shape. This process involves local stretching and rolling of the nanotube, which was otherwise fixed on the substrate via the van der Waals force, resulting in the development of extremely localized strains along the length of the CNT. Although local strain in nanotubes has previously been studied using AFM and transmission electron microscopy [33] , TERS microscopy is the only optical technique that can provide images of such local structural distribution of nanomaterials in nanoscale through Raman spectral analysis. Further, it is interesting to note that when a straight CNT is manipulated into a shape involving local curvature, the atomic arrangements on the inner and outer surfaces of the curved area are modified compared with the straight area. This leads to a local breakdown in symmetry and hence the selections rules of Raman scattering are relaxed in the vicinity of the local curvature, allowing forbidden Raman modes to become visible there. This can be clearly seen in TERS measurements, as new Raman modes start to appear within the length of a few nanometres around the curved area. The combination of our manipulation and high-resolution characterization techniques opens paths for the development of well-controlled CNT-based devices with proper characterization of their performances. The methods are well suited for a variety of applications in optical, electronic, mechanical or bio-related usage of CNTs. However, we believe a careful investigation of strain-induced Raman response is required before this technique can be utilized for other materials, as Raman signatures of strain are strongly material dependent. Manipulation of CNTs to induce local strains As schematically demonstrated in Fig. 1a , we can draw any desired shape from nanotubes, for example, alphabets, by utilizing our contact-mode-based AFM-tip-dragging technique. At the same time, we can also image the dragged nanotube using tapping-mode operation of the AFM, as shown in Fig. 1b , where the nanotubes are not dragged any further. Using the same technique, we prepared a specifically designed sample that has the shape of the word ‘CNT’ ( Fig. 2a–c ). This sample was prepared from a single-walled nanotube lying straight on the substrate, which was dragged from different points to attain the said shape. To obtain two-dimensional TERS images, we raster-scanned a metal-coated tip over the sample in the entire image area shown in Fig. 2a,b , and simultaneously measured locally enhanced Raman spectra around the high-frequency G-band vibrational mode (G + -mode) right under the tip apex. As shown in Fig. 3 , we could clearly observe the enhanced G + -mode only when the tip was located on the nanotube, whereas the far-field intensity of the G + -mode was very weak when the tip was away from the nanotube. We observed no G + -mode when we measured TERS at a location far from the sample (where the sample was outside the diffraction-limit area), which also guaranteed that there was no carbonaceous contamination on the tip. To obtain pure near-field images, we subtracted the weak far-field background in Fig. 2a,b so that only near-field signal remained visible and the background appeared black in the images. Figure 2a shows a TERS image of the sample constructed from the peak positions of the G + -mode, which has a spatial resolution better than 20 nm, about 25 times finer than the value achievable under the diffraction limit of light (excitation wavelength is 488 nm). 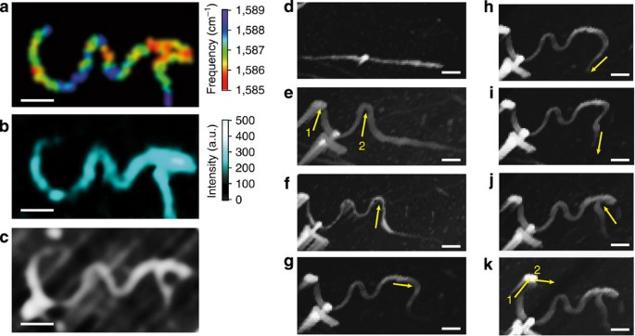Figure 2: Colour-coded nano-Raman imaging of an AFM-manipulated CNT. (a) Two-dimensional colour image of a nanotube manipulated into the shape of the word ‘CNT’. This image was constructed by colour coding the frequency position of G+-mode in TERS spectra. The colour variation shows strain distribution along the nanotube at high spatial resolution. For comparison, TERS images of the same sample were constructed from (b) the intensity of G+-mode and (c) simultaneously obtained AFM topography. (d–k) AFM images showing intermediate steps during the fabrication of the ‘CNT’-shaped sample. Yellow arrows indicate the dragging directions in each step. Scale bars, 100 nm (a–k). The colour variation in this figure corresponds to the local peak position and represents the local variation of strain along the length of the nanotube (explained in more detail later). For comparison, Fig. 2b shows a TERS image constructed from the intensity of Raman peak, where the intensity at each point represents the maximum value obtained at corresponding frequencies plotted in Fig. 2a . Figure 2c shows an AFM image of the same sample. The AFM image in Fig. 2c was obtained simultaneously with the TERS image in Fig. 2b utilizing the same tip (silver coated, with apex size ~25 nm); thus, the spatial resolution in this AFM image is not as high as usual AFM images taken with sharp silicon tips. Both images in Fig. 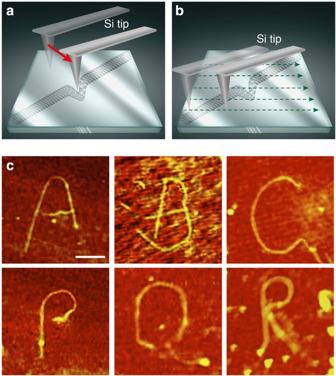2b,c show the physical existence of nanotube manipulated in the shape of the word ‘CNT’. Figure 1: Manipulation of CNTs by an AFM tip. (a) An illustration showing the manipulation scheme. A straight isolated CNT lying on a glass substrate is locally dragged by the sharp apex of an AFM tip, as the tip scans along a straight line in a contact-mode operation with a constant tip-applied force of 20 nN. (b) An illustration showing AFM imaging of a manipulated CNT. The imaging is performed in tapping-mode operation, where there is no more manipulation of the CNT during the imaging process. (c) Some examples of manipulated CNTs, where the CNTs take the shapes of alphabets. Scale bar, 100 nm. Figure 1: Manipulation of CNTs by an AFM tip. ( a ) An illustration showing the manipulation scheme. A straight isolated CNT lying on a glass substrate is locally dragged by the sharp apex of an AFM tip, as the tip scans along a straight line in a contact-mode operation with a constant tip-applied force of 20 nN. ( b ) An illustration showing AFM imaging of a manipulated CNT. The imaging is performed in tapping-mode operation, where there is no more manipulation of the CNT during the imaging process. ( c ) Some examples of manipulated CNTs, where the CNTs take the shapes of alphabets. Scale bar, 100 nm. Full size image Figure 2: Colour-coded nano-Raman imaging of an AFM-manipulated CNT. ( a ) Two-dimensional colour image of a nanotube manipulated into the shape of the word ‘CNT’. This image was constructed by colour coding the frequency position of G + -mode in TERS spectra. The colour variation shows strain distribution along the nanotube at high spatial resolution. For comparison, TERS images of the same sample were constructed from ( b ) the intensity of G + -mode and ( c ) simultaneously obtained AFM topography. ( d – k ) AFM images showing intermediate steps during the fabrication of the ‘CNT’-shaped sample. Yellow arrows indicate the dragging directions in each step. Scale bars, 100 nm ( a – k ). 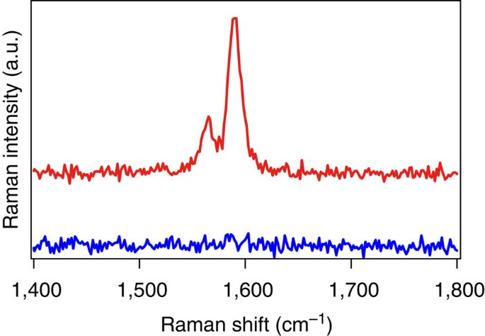Figure 3: TERS spectra of a CNT on the glass substrate. TERS spectrum measured with a silver-coated tip located exactly on the nanotube (red upper plot). TERS spectrum measured with the tip located ~500 nm away from the nanotube directly on the glass substrate (blue lower plot). The absence of any Raman peak in G-band spectral region confirms that there was no carbonaceous contamination on the tip. In addition, we took proper care to keep the sample in clean environment and made sure through Raman measurements that there was no carbonaceous contamination on the substrate as well. Full size image Figure 3: TERS spectra of a CNT on the glass substrate. TERS spectrum measured with a silver-coated tip located exactly on the nanotube (red upper plot). TERS spectrum measured with the tip located ~500 nm away from the nanotube directly on the glass substrate (blue lower plot). The absence of any Raman peak in G-band spectral region confirms that there was no carbonaceous contamination on the tip. In addition, we took proper care to keep the sample in clean environment and made sure through Raman measurements that there was no carbonaceous contamination on the substrate as well. Full size image Figure 2d–k show AFM images of the manipulated CNT, measured during the process of manipulation, which show a sequence of several intermediate manipulation steps where the arrows indicate the direction of dragging in each step. Supplementary Movie 1 shows the intermediate steps in the manipulation process. A random structure seen near the lower left end in the AFM images was a dust particle, which showed no Raman signal within the signature frequency range of CNT, confirming that it was not a carbonaceous material. Therefore, this structure is visible in the AFM images but not seen in the TERS images. It could be a small piece of Ni/Y catalyst used in the arc-discharge synthesis; however, we could not confirm this independently. Analysis of local strain in CNT through TERS nanoimage The dragging method described above introduces local strains in the nanotube by rolling (torsional strain), stretching (tensile strain) or a combination of both [34] , [35] , [36] . TERS imaging, which involves Raman spectroscopy, is the best approach to visualize and analyse these local strains [37] , [38] , [39] , [40] . Raman scattering can even distinguish between torsional and tensile strains in CNTs because the G + -mode around 1,590 cm −1 in Raman scattering shifts towards higher frequency under a torsional strain, whereas it shifts towards lower frequency under a tensile strain [39] , [40] , [41] . In the TERS image shown in Fig. 2a , reddish colours indicate low values of G + -mode frequency, whereas bluish colours indicate high values of G + -mode frequency. Thus, the areas coloured in blue and green in Fig. 2a show the existence of dominant torsional strain, whereas the areas coloured in red and orange indicate dominance of tensile strain. We explain the colours in TERS image, or the step-by-step development of strain in the manipulation process as follows: it can be understood that if the nanotube is pushed from its end, it has a possibility to roll and shift without much elongation, whereas when it is pushed from an inner location far from the free ends, it can go through a significant elongation as well. We can see this in our sample as the two ends of the nanotube, namely, the upper part of the letter ‘C’ and the lower part of the letter ‘T’ show blue and green colours in Fig. 2a , indicating the dominance of torsional strain. The dominance of rolling continues further near the free ends of the nanotube to provide green colour to the left lower part of ‘C’ and to the mid-lower part of ‘T’. The left part of the letter ‘N’ was created from the second push in Fig. 2e , which being located far from the end of the nanotube is expected to dominantly stretch the nanotube in that locality. Some orange and yellow colours can be seen near the upper left part of ‘N’; however, the top area briefly shows blue colour, indicating that the rolling took over the stretching at that point. The lower part of the letter ‘N’ lies between the second push in Fig. 2e and the push in Fig. 2f . It seems that this part of the nanotube has rolled because of the pushes from both sides and resulted in blue-green colours for the lower part of the letter ‘N’. The upper part of the letter ‘T’ was created by the pushes in Fig. 2f,g,j , all of which correspond to locations away from the ends of the nanotube, and hence the upper part for ‘T’ shows red-orange-yellow colours indicating the dominance of stretching. The extremely localized strain developed along the length of the nanotube during the manipulation process can thus be explained and visualized in colours. Spectral analysis of the nature of local strain It can be understood that a CNT would not be much elongated when dragged from its end, and hence the torsional strain should dominate in this case. However, when the nanotube is dragged from an inner location, it could be elongated as well as rolled. The amount of rolling would depend on the frictional forces caused by the van der Waals interaction between the substrate and the nanotube, which actually depends on the physical properties of the nanotube utilized in the experiment, such as the diameter and the chirality. For nanotubes with larger frictional forces, the effect of rolling would surpass the effect of elongation and, hence, the G + -mode may show a higher shift even when the nanotube is dragged from an inner location. To demonstrate and explain this, we prepared a simple sample with a different kind of CNT, where an isolated nanotube was dragged from just two inner locations, marked by points A and B in the AFM image in Fig. 4a . The yellow arrows indicate the directions of dragging. The nanotube used in this sample shows the dominance of rolling even when dragged from an inner location; thus, the frequency of the G + -mode shifts upwards from its original position of about 1,590 cm −1 . We scanned this sample while measuring local TERS spectra at high spatial resolution and constructed three TERS images from Raman intensities of the G + -mode measured at frequencies 1,590, 1,600 and 1,610 cm −1 , which were given three different colours, red, blue and green, respectively. By superimposing these three images, we constructed a colour-coded composite TERS image shown in Fig. 4b . Raman frequencies at 1,600 and 1,610 cm −1 (blue and green, respectively) dominate the bent corners, confirming that the torsional strain was developed around the dragged and bent part of the nanotube. For comparison, Fig. 4c displays an AFM image of a neighbouring non-manipulated straight part of the CNT. 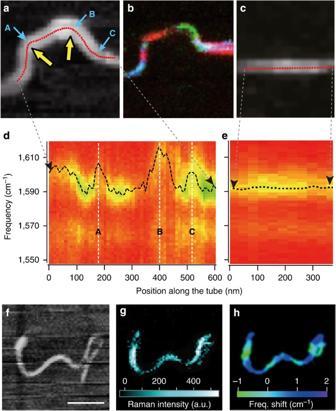Figure 4: Strain induced in CNTs having higher frictional forces. (a) An AFM image of a nanotube, which was dragged along the yellow arrows from two distinct points marked by A and B. (b) A composite TERS image constructed from Raman intensities at three frequencies of 1,590 cm−1(red), 1,600 cm−1(blue) and 1,610 cm−1(green). Frequency-shifted intensity components (blue and green) are dominantly seen at the bent corners. (c) An AFM image of a neighbouring non-manipulated straight part of the sample. (d) The frequency positions of G+-mode in TERS spectra obtained along the length of the manipulated part of the CNT (corresponding to the red dotted path shown ina) and (e) along the non-manipulated neighbouring area (corresponding to the red dotted path shown inc). Raman frequency variation can be seen only in the manipulated part. The vertical dashed lines correspond to the bent points A, B and C inawhere large frequency shifts in the G+-mode are observed. (f) An AFM image of a CNT that was folded into the shape of the letter ‘ω’. (g,h) TERS intensity and frequency-shift images of the G+-mode, respectively, obtained simultaneously with the AFM image. The colour variation inhcorresponds to the variation in local strain along the length of the nanotube. Scale bars, 100 nm (a–c,f). Figure 4d,e show shifts in Raman frequency of G + -mode along the length of the CNT corresponding to the red dotted curves shown in Fig. 4a,c , respectively. In contrast to the previous sample, sharp upshifts corresponding to torsional strain can be seen near the points (points A and B) where the CNT was dragged by the tip apex, although the dragging points lie at inner locations of the nanotube. In addition, upshifts can also be seen at the other corner points, such as at point C in the figure, where the CNT locally rolled even without a push at that location. On the other hand, Fig. 4e confirms that the peak position in the non-manipulated straight part of the CNT remains stable at about 1,591 cm −1 . This result leads us to the conclusion that the nanotube used in this particular experiment had stronger frictional force on the substrate that provided rotational torque to the CNT during manipulation; thus, the resultant strain was a combination of tensile and torsional strains, with torsional strain being stronger in magnitude. Figure 4: Strain induced in CNTs having higher frictional forces. ( a ) An AFM image of a nanotube, which was dragged along the yellow arrows from two distinct points marked by A and B. ( b ) A composite TERS image constructed from Raman intensities at three frequencies of 1,590 cm −1 (red), 1,600 cm −1 (blue) and 1,610 cm −1 (green). Frequency-shifted intensity components (blue and green) are dominantly seen at the bent corners. ( c ) An AFM image of a neighbouring non-manipulated straight part of the sample. ( d ) The frequency positions of G + -mode in TERS spectra obtained along the length of the manipulated part of the CNT (corresponding to the red dotted path shown in a ) and ( e ) along the non-manipulated neighbouring area (corresponding to the red dotted path shown in c ). Raman frequency variation can be seen only in the manipulated part. The vertical dashed lines correspond to the bent points A, B and C in a where large frequency shifts in the G + -mode are observed. ( f ) An AFM image of a CNT that was folded into the shape of the letter ‘ω’. ( g , h ) TERS intensity and frequency-shift images of the G + -mode, respectively, obtained simultaneously with the AFM image. The colour variation in h corresponds to the variation in local strain along the length of the nanotube. Scale bars, 100 nm ( a – c , f ). Full size image Another example is shown in Fig. 4f–h , where another kind of CNT, also showing dominance of torsional strain, was manipulated into the shape of the letter ‘ω’, an AFM image of which is shown in Fig. 4f . Simultaneously obtained intensity image and a frequency-shift image of the sample, constructed from the G + -mode, are shown in Fig. 4g,h . The variation of colour in Fig. 4h indicates variation of strain along the CNT. The dark blue colour corresponding to higher Raman frequency of G + -mode near the corners shows the dominance of torsional strain around those areas. Although the amount of Raman frequency shift for the G + -mode is much smaller compared with that in Fig. 4b , this sample also shows the dominance of torsional strain over the tensile strain even when the dragging point lies at an inner location. Examples in Fig. 4 tell us that depending on the nature of the CNT, either of the two kinds of possible strains can dominate, and our TERS-based microscopic technique can easily evaluate it at an extremely high spatial resolution. Localized breakdown of symmetry Localized strain in CNT modifies the arrangement of carbon atoms in the nanotube. Particularly, if the CNT is locally bent, the inner and the outer curvatures around the bend are different, causing a modified atomic arrangement. This results in the local breakdown of symmetry around the bend, leading to a relaxation in the selection rules of Raman scattering. A previous study has predicted that the relaxation of selection rules by symmetry breakdown in CNT can lead to the observation of as many as six Raman modes in the G-band spectral rage, which are not observed in a relaxed CNT [42] . Thus, besides the shift in the G + -mode shown before, we also expect to observe several new modes in the G-band spectral range around the bent area of the nanotube. For this purpose, we explored the same TERS image shown in Fig. 4b , and investigated the spectral variation along the length of the CNT. The image is reproduced in black-and-white and is shown in Fig. 5a . The radius of curvature at the corner points A, B and C are approximately estimated to be smaller than 100 nm, where we could recognize slight variation in the radii, as shown by the dotted circles around the corners. The spectra obtained from these three points are displayed in Fig. 5b–d , respectively. In addition, a spectrum measured from a point on the non-manipulated straight part of the CNT, marked by D, is shown in Fig. 5e . As expected from the un-manipulated part of the sample, the spectrum in Fig. 5e shows only two peaks corresponding to the usual G − - and G + -modes. However, because of the breakdown in symmetry near the bent corners, the G-band splits into several peaks at all the three points A, B and C. To understand this splitting numerically, we tried to fit the three spectra A, B and C with six Lorentzian peaks, keeping in mind that not all peaks would have non-zero intensity. The best-fitted Lorentzian components are shown by the red dashed curves and the total intensities are shown by the red solid curves in Fig. 5b–d . As expected, smaller radius of curvature causes greater breakdown in symmetry leading to the appearance of larger number of peaks. Six peaks are observed at point B where the radius of curvature is the smallest, whereas only three peaks are observed at point A where the radius of curvature is the largest amongst the three bent corners. The number of peaks, their relative intensities and their frequency positions significantly change when measured at the intervals of 10 nm, confirming that the effect of symmetry breakdown is localized within the vicinity of about 10 nm from the bent corners. Such a highly localized appearance of the symmetry breakdown can only be revealed by our TERS techniques, which cannot be observed in usual far-field Raman measurements. 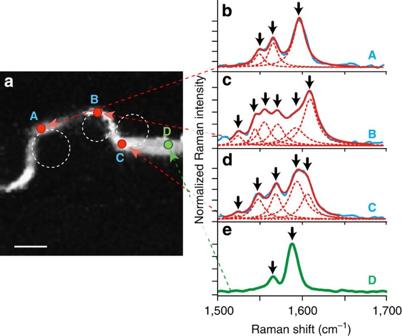Figure 5: Symmetry breakdown induced at the bent corners of the CNT. (a) A TERS intensity image, which is a black-and-white version ofFig. 4b. Three bent corners are marked by the points A, B and C, and the bending curvatures are shown by dotted circles. Point D is marked on the non-manipulated straight part of the CNT. Scale bar, 100 nm (a). (b–e) TERS spectra measured at the points A, B, C and D, indicated ina. The observation of several new modes in the G-band spectral range only at the corners is attributed to the local breakdown in the circumferential symmetry. Figure 5: Symmetry breakdown induced at the bent corners of the CNT. ( a ) A TERS intensity image, which is a black-and-white version of Fig. 4b . Three bent corners are marked by the points A, B and C, and the bending curvatures are shown by dotted circles. Point D is marked on the non-manipulated straight part of the CNT. Scale bar, 100 nm ( a ). ( b – e ) TERS spectra measured at the points A, B, C and D, indicated in a . The observation of several new modes in the G-band spectral range only at the corners is attributed to the local breakdown in the circumferential symmetry. Full size image By utilizing our TERS-based nanoimaging technique, we have successfully demonstrated colour-coded high-resolution nanoimaging of local strain developed along the length of isolated CNTs that were manipulated into various shapes by AFM-tip-dragging method. We confirm an important aspect that the strain developed along the manipulated CNT significantly depends on the intrinsic properties of the nanotubes, such as the chirality and the diameter, which could affect the frictional coefficient. We would also like to mention that we found no noticeable shifts in the D-band mode at 1,334.4 cm −1 or in the radial breathing mode at 166.5 cm −1 of our CNT samples, which indicates that neither the CNTs developed any recognizable defects nor their diameters changed noticeably during this manipulation. Apart from the results shown here with the manipulation of single nanotubes, we also successfully performed the movement of an entire nanotube from one location to another and have written various two-dimensional patterns by manipulating more than one nanotube (some examples can be seen in Fig. 1 ). This manipulation technique is extremely precise and it gives us freedom to utilize a pre-grown nanotube of our choice, and to manipulate them to a shape and a location of our requirement. We have confirmed that these manipulated nanotubes are mechanically stable after the manipulation. Preparation and AFM manipulation of CNTs The single-walled CNTs used in the present study were synthesized by arc discharge and were spin-cast on a glass substrate after proper sonication. We carefully selected those semiconducting nanotubes, which were in good resonance with the excitation wavelength for Raman measurements. For manipulation, almost straight and isolated nanotubes were selected, and the AFM tip operating under the contact-mode configuration was positioned near a specific site of the nanotube. The tip was scanned towards the nanotube along a straight line by maintaining the tip-applied vertical force constant at 20 nN, which dragged the nanotube locally in the direction of tip scanning. Although this dragging resulted in local rolling, stretching and shifting of the nanotube, the nanotubes were well adhered to the substrate and remained stable after the manipulation process was over, as confirmed by AFM images taken under the tapping-mode configuration after the manipulation was finished. To explain our AFM-based manipulation technique that was utilized to prepare the sample, Fig. 1a,b illustrate the dragging of an isolated CNT by an AFM tip during manipulation and the scanning scheme of the AFM tip during topographic imaging after manipulation, respectively. The tip-applied force in the imaging process was 100 times weaker than the tip-applied force during manipulation, which confirmed no further distortion of the sample during the imaging process. After several precisely controlled manipulation steps, the isolated CNTs could be manipulated to any desired shape, for example, to alphabetic shapes, as demonstrated by AFM images in Fig. 1c . The final shapes in Fig. 1c were all stable, confirming that the van der Waals adhesion between the glass substrate and the nanotubes was strong enough to keep the nanotubes stable under the local strains developed by manipulation. This example shows that we can manipulate nanotubes by our AFM-based dragging technique to almost any desired shape and drag them to any required location. TERS imaging of CNTs using a silver-coated tip The SiO 2 tip used in TERS experiments was produced by oxidizing a commercially available AFM-cantilever-tip made of silicon. This oxidized tip was coated with silver by means of a vacuum evaporation method [43] . The oxidization process enabled us to completely evaporate organic compounds adsorbed on the silicon tip, which avoided carbonaceous contamination on probe tips. The TERS signal was measured in the backscattering configuration using an objective lens with a high numerical aperture. We utilized a radially polarized continuous wave laser ( λ =488 nm), which was in good resonance with both the CNTs used in this study as well as with the plasmon excitation of the silver tip. To recognize small shifts in Raman peak, we reduced the spectral resolution to about 0.5 cm −1 by properly selecting the gratings and slit width in our spectrometer. Any possible laser-induced damage was avoided by utilizing very low power of illumination. TERS imaging was performed under the contact-mode operation of tip by raster scanning the sample under a constant tip-applied force of about 0.1 nN. This force was small enough to prevent any dragging, scratching or physical damage of the sample. In addition, this amount of tip-applied force was too small to cause any deformation of the nanotubes during measurement, guaranteeing no Raman spectral shift caused by tip-applied pressure [44] . How to cite this article: Yano, T. et al . Tip-enhanced nano-Raman analytical imaging of locally induced strain distribution in carbon nanotubes. Nat. Commun. 4:2592 doi: 10.1038/ncomms3592 (2013).